Regioselective trifluoromethylation ofN-heteroaromatic compounds using trifluoromethyldifluoroborane activator Many important drugs, agrochemicals and their lead compounds contain trifluoromethyl group(s). Most processes currently used to access trifluoromethyl group-containing molecules are performed by substitution of the carboxy or trichloromethyl groups using hazardous fluorinating reagents under harsh reaction conditions. Cross-coupling reactions between organohalides or boronic acids/esters and trifluoromethylating reagents are also used. Direct C-H trifluoromethylation of organic molecules, however, is the ideal method of introducing trifluoromethyl group(s). Despite the recent advances in C-H trifluoromethylation of N -heteroaromatic compounds, regioselective C-H trifluoromethylation of six-membered heteroaromatic compounds has yet to be achieved. Herein we present a general and reliable method for the synthesis of trifluoromethyl group-containing N -heteroaromatics through highly regioselective addition of a trifluoromethyl nucleophile to pyridine, quinoline, isoquinoline and two or three heteroatom-containing N -heteroaromatic N -oxides activated by trifluoromethyldifluoroborane. The C-H trifluoromethylation proceeds under mild conditions in gram scale with high functional group tolerance. This method will be useful in both laboratory and industrial processes. Organic compounds containing trifluoromethyl (CF 3 ) group(s) are versatile components of drugs, agrochemicals and organic materials. The CF 3 group is highly electron withdrawing, and its introduction can remarkably improve molecular properties, such as lipophilicity, metabolic stability and bioavailability [1] . Therefore, the development of an efficient trifluoromethylation process is currently a main topic in organic synthesis [2] , [3] , [4] , [5] , [6] , [7] , [8] , [9] . Most current processes for accessing CF 3 -containing molecules are performed by carboxy or trichloromethyl group substitution using hazardous fluorinating reagents under harsh reaction conditions [6] . Cross-coupling reactions between organohalides [10] , [11] , [12] , [13] , [14] , [15] , [16] , [17] , [18] , [19] , [20] , [21] , [22] , [23] , [24] or boronic acids (or their esters) [25] , [26] , [27] , [28] , [29] , [30] , [31] , [32] , [33] , [34] and trifluoromethylating reagents are another common approach. Although CF 3 groups can be regioselectively introduced to aromatic rings in cross-coupling reactions, requirement of multiple steps for the preparation of aryl halides and boronic acids/esters and generation of stoichiometric amounts of metal salts decrease synthetic efficiency. To overcome such drawbacks, direct C-H trifluoromethylation recently received much attention; however, examples of aromatic C-H trifluoromethylations are still limited [35] , [36] , [37] , [38] , [39] , [40] , [41] , [42] , [43] , [44] , [45] , [46] . These examples include the following: (1) directing group-assisted palladium [37] , [38] - or silver [39] -catalysed oxidative trifluoromethylation; (2) palladium [40] - or copper [41] -catalysed oxidative trifluoromethylation of heteroaromatic compounds; and (3) radical trifluoromethylation using NaSO 2 CF 3 (ref. 42 ), Zn(SO 2 CF 3 ) 2 (ref. 43 ) or CF 3 SO 2 Cl (ref. 44 ) as the CF 3 source [45] , [46] . The drawback to approach (1), however, is the requirement for directing groups that are not necessary in the target molecules [39] , and in approaches (2) and (3), regioselectivity is generally difficult to control, especially in the case of six-membered heteroaromatic compounds except when using substrates with substituent(s) to block the possible reaction site(s) [40] , [41] , [42] , [43] , [44] , [45] , [46] . Specifically, trifluoromethylation reactions reported by Baran [42] and MacMillan groups [44] are of wide substrate scope. The regioselectivity of those reactions was high in the case of five-membered heteroaromatic substrates. In the case of six-membered heteroaromatic substrates, however, regioselectivity was not satisfactory and mixtures of regioisomers were produced. Among the aromatic compounds containing CF 3 group(s), 2-trifluoromethylpyridine and 2-trifluoromethylquinoline derivatives are especially useful for agrochemicals and drugs. Picoxystrobin [6] and mefloquine [6] are typical examples. We envisioned that regioselective trifluoromethylation of pyridines and quinolines would be possible through dearomatizing nucleophilic addition of the CF 3 group to electrophilically activated N -heteroaromatics, followed by re-aromatization [47] , as an alternative approach to approaches (1), (2) and (3) mentioned above. Here we report a general, regioselective method for the synthesis of CF 3 -containing pyridine, quinoline and isoquinoline derivatives, and other N -heteroaromatics containing two or three heteroatoms, through C-H trifluoromethylation. N -Heteroaromatic N -oxides activated by trifluoromethyldifluoroborane (BF 2 CF 3 ), which are readily prepared, stable and storable, are used as substrates. Non-hazardous, widely used trifluoromethyltrimethylsilane (Me 3 SiCF 3 ) is used as a nucleophilic trifluoromethylating reagent. Trifluoromethylation proceeds under mild conditions even in gram scale and with high functional group tolerance. The present trifluoromethylation reaction can be regarded as a complementary method of the previous ones. DFT calculations N -oxidation and O -acylation or -sulphonylation of the resulting N -oxides are a well-established method for activating N -heteroaromatics as electrophiles [48] . When this method is applied to trifluoromethylation of pyridine derivatives, however, the reaction does not proceed at all. To more efficiently decrease the LUMO level of pyridine-derived substrates, we selected highly Lewis acidic boranes as activators. Theoretical calculations suggest that the LUMO levels of BF 3 and BF 2 CF 3 complexes of pyridine N -oxide are significantly lower than those of O -acyl and -sulphonyl pyridine N -oxides ( Fig. 1 , compounds G and H ). Therefore, BF 2 CF 3 complexes were selected as substrates for C-H trifluoromethylation. 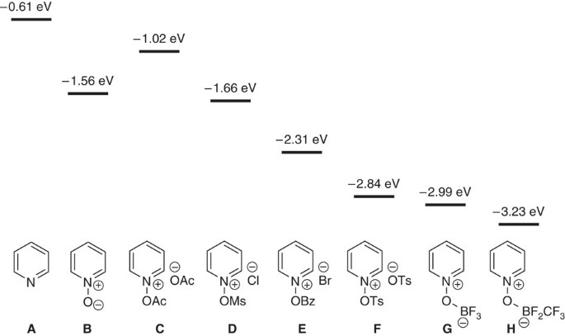Figure 1: Comparison of LUMO levels of several pyridine derivatives. B3LYP/6-31G* for (A); B3LYP/6-31+G* for (B–D,F–H); B3LYP/LAV3P+* for (E). Figure 1: Comparison of LUMO levels of several pyridine derivatives. B3LYP/6-31G* for ( A ); B3LYP/6-31+G* for ( B – D , F – H ); B3LYP/LAV3P+* for ( E ). Full size image Preparation of quinoline N -oxide–BF 2 CF 3 complex Because quinolines are more reactive aromatic compounds than pyridines, we began our optimization using quinoline N -oxide–BF 2 CF 3 complex 2a . Treatment of K[BF 3 CF 3 ] (Tokyo Chemical Industry) with BF 3 ·OEt 2 in dichloromethane at 25 °C for 20 min and subsequent reaction of the thus-generated BF 2 CF 3 ·OEt 2 (refs 49 , 50 ) with quinoline N -oxide ( 1a ) for 1 h afforded quinoline N -oxide–BF 2 CF 3 complex 2a in 90% isolated yield ( Fig. 2 ). Complex 2a and other related molecules were stable under aqueous workup and silica gel column chromatography, and could be stored for at least 3 months without concern regarding exposure to water and oxygen [51] . 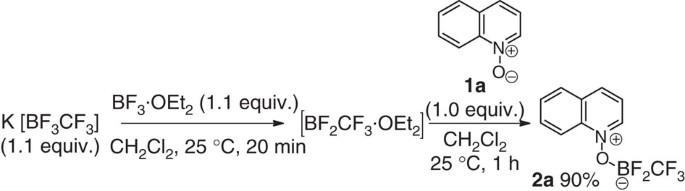Figure 2: Preparation of compound 2a. Formation of quinolineN-oxide–BF2CF3from the correspondingN-oxide. Figure 2: Preparation of compound 2a. Formation of quinoline N -oxide–BF 2 CF 3 from the corresponding N -oxide. Full size image Optimization of reaction conditions Non-hazardous, widely used Me 3 SiCF 3 ( 3 ) was selected as the trifluoromethylating reagent to generate a reactive CF 3 nucleophile by treatment with a fluoride anion. Studies of fluoride salts, such as KF, CsF and n Bu 4 NF, in the reaction between 2a and 3 revealed CsF as the most effective fluoride anion source. Investigation of the amount of CsF, concentration and several solvents indicated that the use of 3.0 equivalents of CsF and ethyl acetate (0.10 M) was optimal ( Table 1 ). Optimization of the temperature, reaction time and the amount of 3 , and addition of MS4A led to an improved yield of 4a : reaction of 2a with Me 3 SiCF 3 ( 3 ) in the presence of CsF at 25 °C for 1 h and then 60 °C for 4 h gave 2-trifluoromethylquinoline ( 4a ) in 91% yield ( Fig. 3 ). This reaction proceeded with high regioselectivity and no other possible regioisomers were detected. When the quinoline N -oxide–BF 3 complex was used, 4a was obtained in less satisfactory yield (45%). The difference in the reactivity between BF 2 CF 3 complex 2a and the corresponding BF 3 complex can be explained by the difference in their LUMO levels ( Fig. 1 ). Table 1 Optimization of reaction conditions. 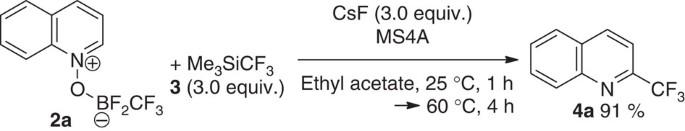Figure 3: Trifluoromethylation of 2a. Optimized conditions for the introduction of the CF3group. Full size table Figure 3: Trifluoromethylation of 2a. Optimized conditions for the introduction of the CF 3 group. Full size image Substrate scope We then investigated the scope of the trifluoromethylation of various N -heteroaromatic compounds ( Table 2 ). The reaction proceeded with high substrate generality and functional group tolerance using several quinoline N -oxide–BF 2 CF 3 complexes bearing electron-donating and -withdrawing groups, giving 2-trifluoromethylquinolines 4b - 4k in excellent yields. Benzo[ h ]quinoline, phenanthridine, and isoquinoline derivatives were also competent substrates, affording 4l - 4n in good to excellent yields. The pyridine derivatives were generally less reactive for nucleophilic addition compared with the corresponding quinoline derivatives. The desired 2-trifluoromethylpyridines 4o - 4v were nevertheless produced in good yields under the developed conditions. In all entries except for acridine-derivative 2w , the trifluoromethylation reaction proceeded exclusively at the carbon adjacent to the nitrogen atom, and regioisomers were not observed by 1 H NMR and GC–MS analyses of the crude products. In the case of acridine N -oxide–BF 2 CF 3 complex 2w , trifluoromethylation occurred exclusively at the 9-position to give 4w . In the cases of heteroaromatic substrates containing two or more heteroatoms, the trifluoromethylated products 4x - 4z and 4A - 4C were obtained with exclusively high regioselectivity as well. Trifluoromethylation reaction did not proceed in the case of five-membered N -heteroaromatic compounds such as imidazole derivatives (for the structures, see the Supplementary Fig. 229 ). Table 2 Trifluoromethylation reactions of several quinoline, isoquinoline and pyridine N -oxide–BF 2 CF 3 complexes 2*. Full size table Gram-scale reaction The reaction can be performed in gram scale. Treatment of 2.38 g of 2d with a mixture of Me 3 SiCF 3 and CsF produced 1.68 g of 4d in 91% yield. The yield of 4d in gram scale was comparable with that shown in Table 1 (74.4-mg scale). Sequential operation without isolation of the intermediates To expand the experimental utility, sequential conversion of 6-chloroquinoline ( 7d ) to 6-chloro-2-trifluoromethylquinoline ( 4d ) was performed without isolation of intermediates 1d and 2d . Oxidation of 6-chloroquinoline ( 7d ) to N -oxide 1d with m -chloroperoxybenzoic acid, successive treatment of 1d with ‘BF 2 CF 3 ’ producing 2d , and the reaction of 2d with Me 3 SiCF 3 and CsF afforded 6-chloro-2-trifluoromethylquinoline ( 4d ) in 69% overall yield ( Fig. 4a ). 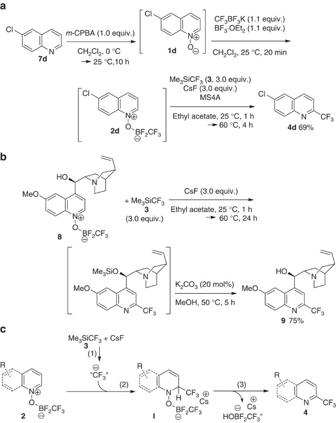Figure 4: Utilities and proposed reaction mechanism of the trifluoromethylation reaction. (a) Sequential operation without isolation of the intermediates. (b) Trifluoromethylation of quinine. (c) Proposed reaction mechanism. Figure 4: Utilities and proposed reaction mechanism of the trifluoromethylation reaction. ( a ) Sequential operation without isolation of the intermediates. ( b ) Trifluoromethylation of quinine. ( c ) Proposed reaction mechanism. Full size image Late-stage trifluoromethylation of quinine Taking advantage of the high functional group tolerance of the present conditions, we examined the application to late-stage trifluoromethylation. Treatment of quinine N -oxide–BF 2 CF 3 complex 8 with a mixture of Me 3 SiCF 3 and CsF, and successive treatment with K 2 CO 3 afforded 2-trifluoromethylated quinine 9 in 75% yield ( Fig. 4b ). The regioselectivity in Fig. 4b was complementary to that reported by Baran and coworkers [42] , in which electrophilic radical trifluoromethylation proceeded at the 7-position of a quinine derivative [41] . The proposed mechanism of the present trifluoromethylation is as follows ( Fig. 4c ; reactions of pyridine and quinoline N -oxides are shown as examples): (1) generation of activated CF 3 nucleophile from Me 3 SiCF 3 and CsF [15] , [16] ; (2) regioselective nucleophilic attack of the formed CF 3 anion to pyridine or quinoline N -oxide–BF 2 CF 3 complex 2 to form dearomatized intermediate I ; and (3) elimination of a borate salt ( Supplementary Table 10 ) to produce 2-trifluoromethylpyridine and -quinoline derivatives 4 . Intermediate I was detected on thin layer chromatography and nuclear magnetic resonance analysis in some reaction conditions and could be isolated by column chromatography on silica gel. Subjecting the isolated intermediate I to the reaction conditions produced 4 in high yield, indicating that product 4 is formed from I ( Supplementary Figs 230 and 231 ; Supplementary Table 9 ). Me 3 SiF, which is formed in the reaction mixture from Me 3 SiCF 3 and CsF, accelerated the re-aromatization step ( Supplementary Fig. 231 ; Supplementary Table 9 ). Because the electron density of the 2-position of the pyridine and quinoline rings is lowest based on the chemical shifts of 1 H and 13 C NMR, trifluoromethylation proceeded selectively at the 2-position. In conclusion, we have developed a regioselective C-H trifluoromethylation reaction of N -heteroaromatic compounds using N -oxide–BF 2 CF 3 complexes as substrates. Trifluoromethyldifluoroborane (BF 2 CF 3 ) electrophilically activated N -heteroaromatics as a powerful Lewis acid. Despite their high reactivity, the N -oxide–BF 2 CF 3 complexes were stable and easy to handle. The reaction proceeded through dearomatizing nucleophilic addition of the trifluoromethyl group to electrophilically activated N -oxide–BF 2 CF 3 complexes, followed by elimination of the borate salt ([HOBF 2 CF 3 ] – ) to recover the aromaticity. Noteworthy characteristics of the developed reaction are as follows: (1) the regioselective trifluoromethylation proceeded without the use of any transition metal catalysts or reagents; (2) the reaction was practical, and could be conducted in gram scale, as well as in a sequential manner starting from non-oxidized N -heteroaromatic compounds, without isolating any intermediates; (3) the reaction proceeded under mild conditions and with high functional group tolerance, as demonstrated by the application to the regioselective trifluoromethylation of quinine. In the previously reported electrophilic radical trifluoromethylation [42] , [44] , regioselectivity control was difficult using six-membered heteroaromatic substrates, whereas regioselectivity was high when using electron-rich five-membered heteroaromatic substrates. In contrast, the present trifluoromethylation proceeded with exclusively high regioselectivity when 6-membered N -heteroaromatics were used as substrates, although the reaction did not proceed in the case of electron-rich five-membered heteroaromatics. Therefore, the present nucleophilic trifluoromethylation reaction can be regarded as a complementary method of the previous radical trifluoromethylation. Combining these two types of reactions, regioselective trifluoromethylation of various heteroaromatic compounds can now be possible. The unique characteristics of N -heteroaromatic N -oxide–BF 2 CF 3 complexes (low LUMO+high stability) will be generally useful for regioselective introduction of other nucleophiles to N -heteroaromatic compounds. General methods For 1H and 13C NMR spectra of compounds in this manuscript, see Supplementary Figs 1–228 . For details of the synthetic procedures, see Supplementary Methods . Preparation of 2d To a mixture of potassium trifluoro(trifluoromethyl)borate (2.15 g, 12.2 mmol, 1.1 equiv.) in dichloromethane (33.0 ml) was added BF 3 ˙OEt 2 (1.51 ml, 12.2 mmol, 1.1 equiv. ), and the mixture was stirred at 25 °C for 20 min. Then, 6-chloroquinoline N -oxide ( 1d , 2.00 g, 11.1 mmol) was added to the reaction mixture and the mixture was stirred at 25 °C for 1 h. After the reaction mixture was diluted with dichloromethane/acetone (1/1), insoluble solid was filtered off, washed with dichloromethane/acetone (1/1) and then the solvent was removed under reduced pressure. The crude product was purified by column chromatography on silica gel (dichloromethane then dichloromethane/acetone=20/1) to give ((6-chloroquinolin-1-ium-1-yl)oxy)difluoro(trifluoromethyl)borate ( 2d , 3.25 g, 98% yield). Synthesis of 4d A mixture of CsF (3.65 g, 24.0 mmol, 3.0 equiv.) and MS4A (800 mg, 100 mg mmol −1 ) was flame-dried under vacuum. After cooling to room temperature, 2d (2.38 g, 8.00 mmol) and ethyl acetate (80 ml) were added. To the mixture, Me 3 SiCF 3 (3.56 ml, 24.0 mmol, 3.0 equiv.) was added dropwise with vigorous stirring. After stirring at 25 °C for 1 h, the mixture was heated at 60 °C for 4 h, and then cooled to room temperature. Insoluble solid was filtered off, washed with ethyl acetate and the solvent was removed under reduced pressure. The crude product was purified by column chromatography on silica gel (hexane/ethyl acetate=15/1) to give 6-chloro-2-(trifluoromethyl)quinoline ( 4d , 1.68 g, 91% yield). How to cite this article : Nishida, T. et al. Regioselective trifluoromethylation of N -heteroaromatic compounds using trifluoromethyldifluoroborane activator. Nat. Commun. 5:3387 doi: 10.1038/ncomms4387 (2014).